Singlet oxygen triplet energy transfer-based imaging technology for mapping protein–protein proximity in intact cells Many cellular processes are carried out by large protein complexes that can span several tens of nanometres. Whereas forster resonance energy transfer has a detection range of <10 nm, here we report the theoretical development and experimental demonstration of a new fluorescence-imaging technology with a detection range of up to several tens of nanometres: singlet oxygen triplet energy transfer. We demonstrate that our method confirms the topology of a large protein complex in intact cells, which spans from the endoplasmic reticulum to the outer mitochondrial membrane and the matrix. This new method is thus suited for mapping protein proximity in large protein complexes. Protein machines carry out almost every major biological process, including DNA replication, gene transcription, protein translation and degradation of RNA and protein [1] . Recently, with the use of global proteomic methods, the number of identified stable protein associations has increased [2] , [3] , [4] . To gain insight into molecular mechanisms, forster resonance energy transfer (FRET) has been widely used to characterize protein–protein interactions [5] , [6] . FRET is based on the interaction between a donor’s emission and an acceptor’s absorption dipole moments. Because the dipole–dipole interaction decays rapidly over distance, FRET has a detection range of <10 nm, which limits its application in multi-protein complexes that span several tens of nanometres (nm) in diameter. To overcome FRET’s distance limitation, we have developed a new method of molecular imaging: singlet oxygen triplet energy transfer (STET). STET is based on a photosensitizing singlet oxygen generator (SOG) and a fluorescent singlet oxygen sensor (SOS). The proximity of protein X to protein Y can be assayed by fusing X to SOG and Y to SOS. Upon illumination, SOG is excited to the first-excited-singlet-state (S 1 ), which crosses to the first-excited-triplet-state (T 1 ) via intersystem crossing. Intersystem crossing is made possible through a spin–orbit interaction that flips the spin of the excited electron, resulting in the non-radiative S 1 →T 1 transition [7] . The SOG at the T 1 state can then convert triplet oxygen ( 3 O 2 ) into singlet oxygen ( 1 O 2 ) through triplet energy transfer [8] , [9] . Reactive 1 O 2 reaching SOS through diffusion reacts with the sensor to alter its fluorescence intensity. Whether or not this reaction is limited by singlet oxygen diffusion depends on the reaction rate of the specific SOS with singlet oxygen. Regardless of this, the fluorescence-intensity change rate of SOS is dependent on the amount of 1 O 2 it senses per time (that is, the flux of 1 O 2 ), which is a function of distance: the closer the two proteins are, the faster the fluorescence intensity of SOS changes. Here, we define the fluorescence-intensity change rate of SOS as a STET signal, which reports protein proximity. Because 1 O 2 has been estimated to diffuse at least several tens of nanometres in cells within its half-life [10] , [11] , STET is expected to function over a greater distance (>30 nm) than FRET. We use a previously engineered infrared fluorescent protein (IFP1.4) as SOS [12] , and a small singlet oxygen photosensitizer (miniSOG) as a SOG [13] . We first demonstrate that IFP1.4 specifically senses singlet oxygen, but not other reactive oxygen species (ROS), including hydrogen peroxide (H 2 O 2 ), superoxide and a hydroxyl radical. We also show that this specific sensitivity of IFP1.4 to singlet oxygen is mainly owing to its chromophore, biliverdin (BV). Next, we confirmed that singlet oxygen is involved in STET, while other ROS are not. We then demonstrate that STET signal is dependent on the distance between the sensor and the generator, by using linkers of different lengths between SOG and SOS. To demonstrate STET in intact cells, we choose a large protein complex that spans from the endoplasmic reticulum (ER) to the mitochondrial outer membrane (MOM) and the matrix. We show that the STET signal confirms the topology of the complex. Finally, our STET experiment suggests that a mitochondrial inner membrane (MIM) protein that has previously been shown to genetically interact with other components of the machinery is likely to be part of the complex. Concept of STET To realize the concept of STET ( Fig. 1a ), we made use of two genetically encoded protein tags, miniSOG and IFP1.4, which require no exogenous cofactors. miniSOG is green fluorescent and generates 1 O 2 when illuminated with blue light (450–490 nm) [13] . IFP1.4 absorbs maximally at 684 nm and emits at 710 nm [12] . Thus, there is little spectral overlap between SOG and SOS. Both SOG and SOS are monomeric, making it unlikely for them to alter the stoichiometry of tagged proteins, which is necessary for the correct assembly of complexes. 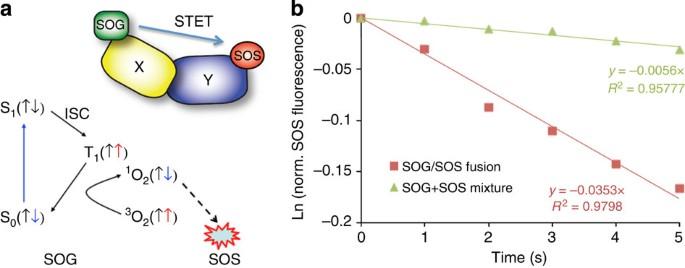Figure 1: Development of singlet oxygen triplet energy transfer-based technology. (a) Schematic diagram showing physical principles of STET. (b) Natural logarithm of normalized fluorescence intensity of SOS over time under blue-light illumination in the fusion (1 μM) versus mixture of SOG and SOS (1 μM each). Figure 1: Development of singlet oxygen triplet energy transfer-based technology. ( a ) Schematic diagram showing physical principles of STET. ( b ) Natural logarithm of normalized fluorescence intensity of SOS over time under blue-light illumination in the fusion (1 μM) versus mixture of SOG and SOS (1 μM each). Full size image To demonstrate the dependence of STET on protein proximity, we compared the STET signals of a purified fusion protein of SOG and SOS with that of a mixture of individually purified SOG and SOS. Constant blue-light illumination (488 nm) of the fusion protein, which produces 1 O 2 from SOG, caused a decrease in the infrared fluorescence intensity of SOS ( Fig. 1b ). The natural logarithm of normalized SOS fluorescence intensity at different time points fits the linear equation y =− αt , suggesting that SOS senses a constant flux of 1 O 2 . In other words, constant illumination of SOG creates a steady state of concentration gradient of 1 O 2 . We calculated the STET signal from the slope ( α ) of the fitted equation (details in Methods). Importantly, the SOG/SOS fusion protein has a significantly larger STET signal than the mixture ( Fig. 1b ), demonstrating that STET reflects protein proximity (see further characterizations in the following sections). Reaction of IFP1.4 with ROS To demonstrate that IFP1.4 is a SOS, we reacted IFP1.4 with various ROS ( Fig. 2 ). For the reaction with superoxide, we used two different sources of superoxide: potassium superoxide (KO 2 ) ( Fig. 2b ); and superoxide generated by the reaction of xanthine oxidase and xanthine ( Fig. 2c ) [14] . On addition of superoxide from each source, the fluorescence of IFP1.4 did not change ( Fig. 2b,c , Methods). On the other hand, the fluorescence of hydrocyanine 3 (a fluorogenic probe for superoxide) increased significantly upon reaction with KO 2 ( Supplementary Fig. 1a ). Next, we reacted IFP1.4 with H 2 O 2 , which also had no effect on the fluorescence of IFP1.4 ( Fig. 2d ). To test whether the hydroxyl radical could affect the IFP1.4’s fluorescence, we used Fenton’s reaction to generate the hydroxyl radical by reacting H 2 O 2 with Fe 2+ . However, the fluorescence of IFP1.4 did not change ( Fig. 2e ). Finally, we reacted IFP1.4 with singlet oxygen. We used two sources of singlet oxygen: (1) reacting H 2 O 2 with sodium hypochlorite (NaClO) ( Fig. 2g ); (2) perinaphthenone, an efficient singlet oxygen photosensitizer, which generates singlet oxygen upon blue-light excitation ( Fig. 2h ) [15] . IFP1.4 reacted strongly with both sources of singlet oxygen, based on the significant change of its fluorescence ( Fig. 2g,h ). As a control, sodium chlorite has no effect on IFP1.4’s fluorescence ( Fig. 2f ). These results demonstrate that IFP1.4 senses singlet oxygen but not other ROS including superoxide, H 2 O 2 and hydroxyl radical. We therefore conclude that IFP1.4 is a specific SOS. 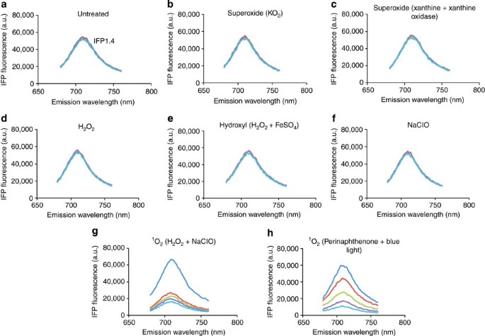Figure 2: Reaction of IFP1.4 with reactive oxygen species. Fluorescence spectra of IFP1.4 reacted: (a) without ROS; (b) with superoxide from KO2; (c) with superoxide generated by xanthine and xanthine oxidase; (d) with hydrogen peroxide; (e) with hydroxyl radical; (f) with sodium hypochlorite; (g) with singlet oxygen generated from hydrogen peroxide and sodium hypochlorite; and (h) with singlet oxygen photo-generated from perinaphthenone. Different colours of the lines refer to time after reaction (a–g) or exposure time (h): blue (0 min); red (5 min); green (10 min); purple (15 min); cyan (20 min). Figure 2: Reaction of IFP1.4 with reactive oxygen species. Fluorescence spectra of IFP1.4 reacted: ( a ) without ROS; ( b ) with superoxide from KO 2 ; ( c ) with superoxide generated by xanthine and xanthine oxidase; ( d ) with hydrogen peroxide; ( e ) with hydroxyl radical; ( f ) with sodium hypochlorite; ( g ) with singlet oxygen generated from hydrogen peroxide and sodium hypochlorite; and ( h ) with singlet oxygen photo-generated from perinaphthenone. Different colours of the lines refer to time after reaction ( a – g ) or exposure time ( h ): blue (0 min); red (5 min); green (10 min); purple (15 min); cyan (20 min). Full size image We then tried to explain why IFP1.4 specifically senses singlet oxygen. It is known that ROS including H 2 O 2 , superoxide, hydroxyl radical and singlet oxygen can generally react with proteins. Our data showing that IFP1.4 only senses singlet oxygen thus suggest that the specificity may come from the chromophore of IFP1.4, BV. To test this hypothesis, we reacted BV with various ROS and monitored its absorbance over time ( Fig. 3 ). First, there was no change in the absorbance spectra of BV when we added KO 2 ( Fig. 3b ), similar to the no-ROS control ( Fig. 3a ). This suggests that BV did not react with superoxide. Similarly, we observed no absorbance change in BV when it was mixed with H 2 O 2 solution ( Fig. 3c ) or the Fenton’s reagent ( Fig. 3d ), suggesting that BV did not react with H 2 O 2 or hydroxyl radical. Finally, we reacted BV with perinaphthenone under blue-light excitation and detected a significant decrease in the absorbance spectra ( Fig. 3e ), indicating that BV reacted readily with singlet oxygen. Interestingly reaction of BV with singlet oxygen has been previously reported [16] . Our results demonstrate that BV reacts specifically with singlet oxygen but not any other ROS examined here. 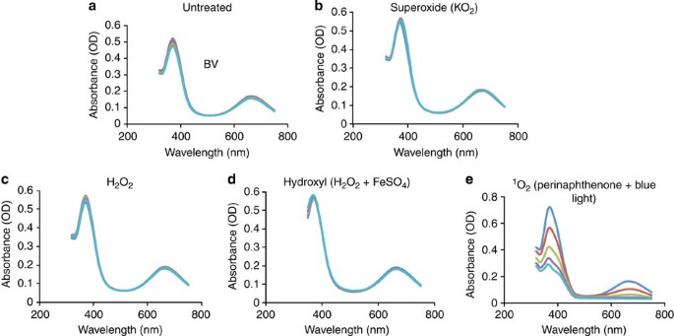Figure 3: Reaction of biliverdin with reactive oxygen species. Absorbance spectra of biliverdin reacted: (a) without ROS; (b) with superoxide from KO2; (c) with hydrogen peroxide; (d) with hydroxyl radical; and (e) with singlet oxygen photo-generated from perinaphthenone. Different colours of the lines refer to time after reaction (a–d) or exposure time (e): blue (0 min); red (5 min); green (10 min); purple (15 min); cyan (20 min). Figure 3: Reaction of biliverdin with reactive oxygen species. Absorbance spectra of biliverdin reacted: ( a ) without ROS; ( b ) with superoxide from KO 2 ; ( c ) with hydrogen peroxide; ( d ) with hydroxyl radical; and ( e ) with singlet oxygen photo-generated from perinaphthenone. Different colours of the lines refer to time after reaction ( a – d ) or exposure time ( e ): blue (0 min); red (5 min); green (10 min); purple (15 min); cyan (20 min). Full size image Furthermore, reaction of IFP1.4 with singlet oxygen resulted in decrease of the absorbance peak (684 nm) of IFP1.4 ( Supplementary Fig. 1b ). Since the absorbance peak of free BV is 660 nm, and we did not observe a blue shift of the IFP1.4’s absorbance peak, our data suggest that reaction of IFP1.4 with singlet oxygen does not cause release of bound BV from the protein. Thus the loss of IFP1.4’s fluorescence upon reaction with singlet oxygen is caused by reaction of singlet oxygen with BV. On the basis of these results, we conclude that the specific sensitivity of IFP1.4 towards singlet oxygen is mainly due to the reaction of its chromophore with singlet oxygen. Although reaction of other ROS with the protein has no apparent effect on the fluorescence of IFP1.4, we cannot exclude the possibility, despite its unlikelihood, that reaction of singlet oxygen with residues in the protein may also contribute to the change of IFP1.4’s fluorescence. Effect of various ROS quenchers on STET The demonstration of IFP1.4 as a specific SOS strongly suggests that singlet oxygen is involved in producing the STET signal. To further confirm this, we tried to quench STET using various ROS quenchers ( Fig. 4 ). On addition of superoxide dismutase (SOD), a superoxide quencher, to the solution of IFP1.4 and miniSOG, we did not observe any effect on STET ( Fig. 4c,f ). The STET signal in the presence of SOD is similar to the control without any quencher ( Fig. 4b,f ). Addition of catalase, a H 2 O 2 quencher, did not affect STET either ( Fig. 4d,f ). Finally, we tested whether a singlet oxygen quencher would quench STET. Because sodium azide is known to quench the triplet-excited state of flavin mononucleotide [17] (the chromophore of miniSOG), we decided to use glutathione (GSH). GSH has been shown to react and quench singlet oxygen efficiently, forming various products including GSH disulphide, GSH sulphoxide, GSH sulphonate and GSH sulphinate [18] . On addition of GSH, STET is completely quenched ( Fig. 4e,f ) to a level similar to the control without SOG ( Fig. 4a,f ). These results confirm that singlet oxygen is involved in STET, whereas other ROS including superoxide, H 2 O 2 and hydroxyl radical are not. 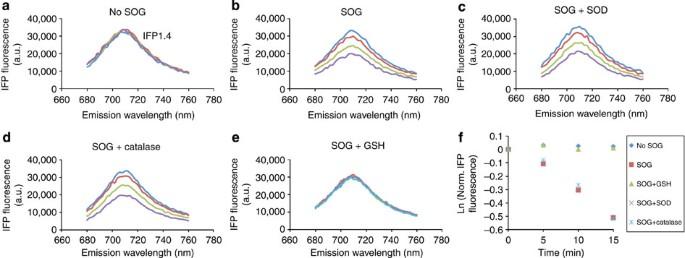Figure 4: Quenching of STET with various ROS quenchers. (a) Fluorescence spectra of IFP1.4 without SOG. (b) Fluorescence spectra of IFP1.4 in the presence of SOG. (c–e) Fluorescence spectra of IFP1.4 in the presence of SOG and (c) superoxide quencher SOD; (d) hydrogen peroxide quencher catalase; and (e) singlet oxygen quencher glutathione (GSH). (f) Natural logarithm of normalized fluorescence intensity of IFP1.4 over time under blue-light illumination. Different colours of the lines refer to time after reaction (a–e): blue (0 min); red (5 min); green (10 min); purple (15 min); cyan (20 min, paneleonly). Figure 4: Quenching of STET with various ROS quenchers. ( a ) Fluorescence spectra of IFP1.4 without SOG. ( b ) Fluorescence spectra of IFP1.4 in the presence of SOG. ( c – e ) Fluorescence spectra of IFP1.4 in the presence of SOG and ( c ) superoxide quencher SOD; ( d ) hydrogen peroxide quencher catalase; and ( e ) singlet oxygen quencher glutathione (GSH). ( f ) Natural logarithm of normalized fluorescence intensity of IFP1.4 over time under blue-light illumination. Different colours of the lines refer to time after reaction ( a – e ): blue (0 min); red (5 min); green (10 min); purple (15 min); cyan (20 min, panel e only). Full size image Dependence of STET on distance To further demonstrate that STET is dependent on the distance between SOG and SOS, we made three constructs that connect SOG and SOS with linkers of various lengths: (1) 5 amino acids (aa); (2) 73 aa; and (3) 133 aa. Indeed, the fusion protein of SOG and SOS with the shortest linker produced the largest STET signal, whereas the fusion protein with the longest linker had the smallest STET signal ( Fig. 5 ). The fusion protein with the intermediate linker length resulted in an intermediate STET signal. Therefore, our results demonstrate that STET is dependent on the distance between SOG and SOS. 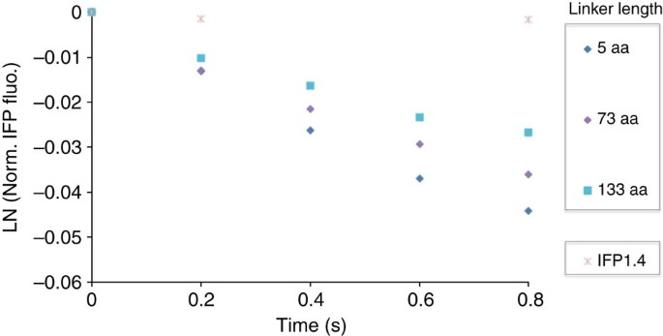Figure 5: Dependence of STET on distance between SOG and SOS. Natural logarithm of normalized fluorescence intensity of IFP1.4 over time under blue-light illumination. Figure 5: Dependence of STET on distance between SOG and SOS. Natural logarithm of normalized fluorescence intensity of IFP1.4 over time under blue-light illumination. Full size image We also examined the dependence of STET on the concentration of SOG. In this case, we mixed different concentrations of SOG with SOS. Upon increasing the concentration of SOG from 0.3 to 10 μM, the STET signal increased linearly ( Fig. 6 ). 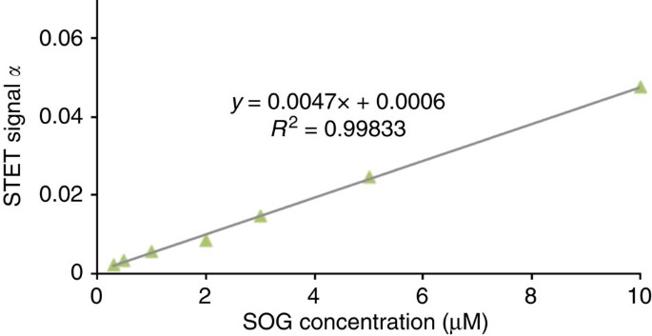Figure 6: Dependence of STET on SOG concentration. The STET signalαis obtained from fitting the natural logarithm of normalized SOS fluorescence to a linear equationy=−αt. The STET signal versus concentration is fitted by a linear line (dashed). Figure 6: Dependence of STET on SOG concentration. The STET signal α is obtained from fitting the natural logarithm of normalized SOS fluorescence to a linear equation y =− αt . The STET signal versus concentration is fitted by a linear line (dashed). Full size image Demonstration of STET in intact cells To demonstrate STET in intact cells, we mapped protein proximity within a large protein complex. The ER and mitochondria in Saccharomyces cerevisiae are physically tethered by the ER-mitochondria encounter structure (ERMES) [19] , which spans ~\n40 nm and is composed of the ER transmembrane protein Mmm1, the two MOM proteins Mdm34 and Mdm10 and the cytosolic protein Mdm12. In addition, the mitochondrial nucleoid protein Mgm101 co-immunoprecipitates with ERMES [20] and partially co-localizes with Mmm1 by fluorescence [21] . Because replicating mitochondrial DNA (mtDNA) co-localizes with Mmm1 (refs 21 , 22 ) (whereas non-replicating mtDNA does not), it has been proposed that mtDNA replication is regulated by the large protein complex that includes ERMES and Mgm101 and spans three membranes from the ER to the mitochondrial matrix [21] . Because ERMES has a known topology across inter-organelle membranes, we elected to use STET to analyse its structure ( Fig. 7a ). 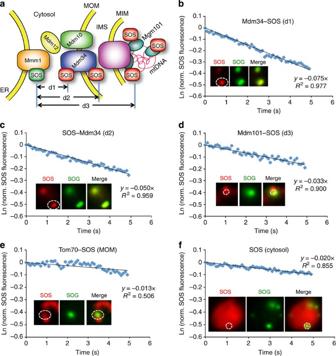Figure 7: STET reports protein proximity in intact cells. (a) Schematic diagram showing topology of the ERMES complex. (b–f) Natural logarithm of normalized fluorescence intensity of SOS (region within white circle in the inset) over time under blue-light illumination (488 nm) with SOG attached to the cytosolic face of Mmm1 and SOS to: the cytosolic face of Mdm34 (b); the IMS face of Mdm34 (c); the Mgm101 in the matrix (d); the cytosolic face of Tom70 (e); and the cytosol (that is, free SOS) (f). IMS: intermembrane space. (MOM, mitochondrial outer membrane. Blue diamond indicates measured data point. Solid line indicates linear fit of the data. Insets show fluorescence images at time=0 s). Figure 7: STET reports protein proximity in intact cells. ( a ) Schematic diagram showing topology of the ERMES complex. ( b – f ) Natural logarithm of normalized fluorescence intensity of SOS (region within white circle in the inset) over time under blue-light illumination (488 nm) with SOG attached to the cytosolic face of Mmm1 and SOS to: the cytosolic face of Mdm34 ( b ); the IMS face of Mdm34 ( c ); the Mgm101 in the matrix ( d ); the cytosolic face of Tom70 ( e ); and the cytosol (that is, free SOS) ( f ). IMS: intermembrane space. (MOM, mitochondrial outer membrane. Blue diamond indicates measured data point. Solid line indicates linear fit of the data. Insets show fluorescence images at time=0 s). Full size image To demonstrate whether STET can map the topology of ERMES, we created three yeast strains that express the following: (i) SOG fused to the cytosolic face of Mmm1 (Mmm1–SOG), and SOS fused to the cytosolic face of Mdm34 (Mdm34–SOS); (ii) Mmm1–SOG, along with SOS fused to Mdm34 facing the intermembrane space (SOS–Mdm34); and (iii) Mmm1–SOG and SOS fused to Mgm101 in the matrix (Mgm101–SOS). Another two yeast strains were created as controls: (iv) Mmm1–SOG and SOS fused to the cytosolic face of the MOM protein Tom70; and (v) Mmm1–SOG and free SOS in the cytosol. Tom70 is part of the translocase of the outer membrane complex [23] , and is not associated with Mmm1. We illuminated yeast cells at 488 nm to photo-excite SOG, producing 1 O 2 and green fluorescence; simultaneous illumination at 642 nm was also done to photo-excite SOS. The green (525±25 nm) and infrared fluorescence (705±36 nm) were collected at 100 ms per frame. First, we observed punctate fluorescent structures in the above strains ( Fig. 7b–f inset). Similar punctate structures were previously seen with enhanced green fluorescent protein (GFP) labelling of the complex, with each punctum representing one junction between ER and mitochondrion [19] . Furthermore, the green fluorescence of Mmm1–SOG: (1) overlaps with the infrared fluorescence of SOS fused to Mdm34, consistent with previous results using GFP and red fluorescent proteins [21] ; and (2) partially overlaps with SOS fluorescence of the Mgm101–SOS, which was observed previously with GFP and red fluorescent protein labelling [20] . These results indicate that SOG and SOS have no or little effect on assembly of the protein complex. Second, upon blue-light excitation of SOG, fluorescence intensity of SOS decreased in response to 1 O 2 produced by SOG, as: (1) the STET signal of Mdm34–SOS (facing the cytosol) is the greatest ( Fig. 7b ; Supplementary Fig. 2 ), 0.082±0.006 s −1 averaged from 5 puncta; (2) the STET from Mmm1–SOG to SOS–Mdm34 is smaller ( Fig. 7c ; Supplementary Fig. 3 ), 0.052±0.005 s −1 ; and (3) the STET from Mmm1–SOG to Mgm101–SOS is the smallest among the three strains ( Fig. 7d ; Supplementary Fig. 4 ), 0.037±0.004 s −1 . In the strain expressing Mgm101–SOS, the STET signal was calculated from the region of fluorescence overlap between Mgm101–SOS and Mmm1–SOG (see Methods). The STET signal in the region of non-overlap is smaller (0.023±0.003 s −1 ), presumably reflecting that SOS in this region is several hundred nanometres away from SOG (their non-overlapping fluorescence suggests larger separation than the light diffraction limit, which is 200–300 nm). The differential STET observed in the three strains reflects relative separations between interacting proteins in a cell. In contrast, the control strains show that STET from Mmm1–SOG to Tom70–SOS is 0.020±0.006 s −1 ( Fig. 7e ; Supplementary Fig. 5 ), while STET from Mmm1–SOG to free cytosolic SOS is 0.017±0.004 s −1 ( Fig. 7f ; Supplementary Fig. 6 ). STET signals in these control strains were calculated from the overlapping region of SOS and SOG fluorescence. As expected, STET from the non-interacting protein Tom70 is significantly smaller than that of Mgm101 (the overlapping region), despite the fact that both SOG (ER) and SOS (MOM) are on the cytosolic face. In the absence of SOG, there is little change of SOS fluorescence (<0.006 s −1 ) under the same illumination conditions ( Supplementary Fig. 7 ), suggesting that photobleaching of SOS is negligible. Taken together, the above analysis demonstrates that the STET signal confirms the topology of the large protein complex and that STET works over several tens of nanometres (the size of ERMES is ~\n40 nm), which bridges the imaging gap between FRET (<10 nm) and conventional fluorescence microscopy (>200 nm). Preliminary application of STET We also used STET to evaluate potential components at the MIM, which connects mtDNA to ERMES. Two transmembrane proteins in the MIM, Mdm31 and Mdm32, were previously shown to be functionally important in maintaining mtDNA [24] . However, it is unknown whether they physically link ERMES to Mgm101 and/or mtDNA. Our preliminary results suggest that the MIM protein Mdm32 could be a physical linker, as evidenced by a strong STET signal of 0.054±0.003 s −1 ( Fig. 8 ; Supplementary Fig. 8 ). Nevertheless, further interrogations using genetic and biochemical methods are necessary to confirm our result. 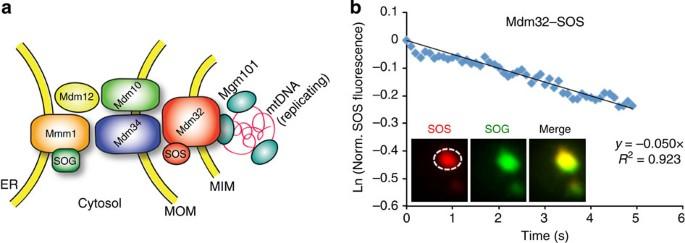Figure 8: STET identifies a potential interacting partner. (a) Proposed schematic diagram showing Mdm32 as the MIM component of the ERMES complex. (b) Natural logarithm of normalized fluorescence intensity of SOS (region within white circle in the inset) over time under blue-light illumination (488 nm) with SOG attached to the cytosolic face of Mmm1 and SOS to Mdm32. (MIM: mitochondrial inner membrane. Blue diamond indicates measured data point. Solid line indicates linear fit of the data. Insets show fluorescence images at time=0 s). Figure 8: STET identifies a potential interacting partner. ( a ) Proposed schematic diagram showing Mdm32 as the MIM component of the ERMES complex. ( b ) Natural logarithm of normalized fluorescence intensity of SOS (region within white circle in the inset) over time under blue-light illumination (488 nm) with SOG attached to the cytosolic face of Mmm1 and SOS to Mdm32. (MIM: mitochondrial inner membrane. Blue diamond indicates measured data point. Solid line indicates linear fit of the data. Insets show fluorescence images at time=0 s). Full size image To overcome the distance limitation of FRET, we have developed and demonstrated a new imaging method, STET, based on the long diffusion distance of singlet oxygen over at least several tens of nanometres in cells. Measuring the exact diffusion distance of singlet oxygen in cells is challenging, though. The diffusion distance depends on the singlet oxygen lifetime and the diffusion coefficient of singlet oxygen in the specific part of the cell. It is challenging to measure both values accurately, although significant advancement has been achieved recently [25] . Although the exact diffusion distance may require further investigation, it seems clear that singlet oxygen can diffuse at least several tens of nanometres in cells within its half-life. Therefore, STET is able to detect protein proximity over much longer distances (>30 nm) than FRET (<10 nm). We have demonstrated that IFP1.4 is a specific SOS by reacting IFP1.4 with different ROS and monitoring its infrared fluorescence. We have further shown that this specificity is due to the specific reactivity of BV, the chromophore of IFP1.4, with singlet oxygen. Although H 2 O 2 , superoxide, and hydroxyl radical are all known to react with proteins—which would change the local environment of the chromophore—it seems that such a potential change does not perturb the electronic structure of BV in IFP1.4. We have also verified that singlet oxygen, but not other ROS, is involved in STET by using different ROS quenchers. This is consistent with the original work of miniSOG [13] , in which miniSOG is designed and shown to efficiently polymerize diaminobenzidine (DAB) to generate electron microscopic (EM) contrast in order to locate proteins of interest in cells at nanometre resolution. It is well known through decades of work that efficient singlet oxygen photosensitizers, such as Eosin, can polymerize DAB [26] . After the publication of miniSOG, two groups have reported that singlet oxygen generation by miniSOG is complicated. Both groups have observed that initially miniSOG photo-produces singlet oxygen inefficiently, with a quantum yield of 0.03±0.01 (ref. 27 ) or 0.030±0.002 (ref. 28 ). Under prolonged irradiation, however, the singlet oxygen generation quantum yield increases significantly (up to 10-fold). To explain the initial small singlet oxygen quantum yield of miniSOG, the two groups have proposed different mechanisms though. On the one hand, Ruiz-Gonzalez et al . [27] attributed the small singlet oxygen quantum yield to ‘a substantial fraction of the nascent 1 O 2 molecules being quenched on their way off the protein’. These authors have proposed that initially, certain residues in the protein quench a significant amount of 1 O 2 , which accounts for the small 1 O 2 quantum yield. After inactivation of those residues, 1 O 2 molecules can efficiently diffuse out of the protein, which explains the irradiation-dependent increase of 1 O 2 quantum yield. On the other hand, Pimenta et al . [28] have proposed a different mechanism and hypothesized that type I chemistry is involved, at the expense of singlet oxygen generation by type II chemistry. These authors have proposed that miniSOG photo-generates H 2 O 2 and superoxide ion. The authors are cautious about this hypothesis and have mentioned caveats in their data, though. Regardless of the disagreement on the possible mechanism for the initially small 1 O 2 quantum yield of miniSOG, both groups agreed and observed that 1 O 2 quantum yield increased significantly over time upon irradiation. As noted by Ruiz-Gonzalez et al . [27] , such irradiation-dependent increase of the quantum yield ‘… may be the reason why miniSOG outperforms other fluorescent proteins reported to date as SOGs’. It is also consistent with the previous observations, as mentioned in the miniSOG paper [13] , that miniSOG can polymerize DAB significantly more efficiently than ReAsH ( 1 O 2 quantum yield 0.024). It seems to us that under the experimental settings for STET and EM applications, miniSOG photo-generates 1 O 2 efficiently. Interestingly, Pimenta et al . [28] observed that even after prolonged irradiation when the 1 O 2 quantum yield increased significantly, photobleaching of miniSOG was not observed, supporting such a notion that miniSOG is ‘activated’ under the EM and STET settings, with no photo-damage during such ‘activation’. We have shown that STET is dependent on distance between SOG and SOS. We have further demonstrated that STET is able to confirm the topology of a large protein complex that spans from the ER to the mitochondrial matrix. For future applications of STET in comparing relative proximity between proteins in a protein complex, we suggest fusing SOG to the same protein and fusing SOS to various interacting partners in order to obtain comparable signals. This is because, as we have demonstrated, the STET signal is linearly proportional to SOG concentration. Using the same SOG fusion will more likely assure similar SOG concentration and thus comparable STET signals among different protein pairs. Furthermore, if SOG expression varies among different samples, we suggest to normalize the STET signal by the SOG fluorescence, which is linearly proportional to the SOG concentration. We also suggest fixing cells to preserve the protein complex since oxidation of residues by singlet oxygen might perturb the topology of a protein complex. Finally, we suggest using constant irradiation so that a steady state of singlet oxygen concentration gradient can be established in cells, which will decrease the heterogeneity of cellular environment since the main quenchers of singlet oxygen in cells have been previously suggested to be certain residues in proteins [10] , [11] , [29] and once those residues are oxidized, a homogenous environment may be established. In summary, we have developed the STET-imaging method, which can be used to detect protein–protein proximity over distances spanning several tens of nanometres. The green and infrared fluorescence of miniSOG and IFP1.4 can first be used to reveal whether potentially interacting proteins of interest are colocalized. If they are colocalized under conventional microscopy, which would suggest that they are within ~\n200 nm range, the users can then easily carry out the STET experiment to estimate the relative distance. The STET method is an alternative but it is not intended to replace other imaging methods such as super-resolution microscopy or electron microscopy. Protein purification SOG (miniSOG in this study), SOS (IFP1.4 in this study) and SOG/SOS fusion proteins were expressed with a C-terminal polyhistidine-tag on a pBAD expression vector (Invitrogen), using TOP10 Escherichia coli (Invitrogen) as the host. Three flexible polypeptide linkers of various lengths in amino acids (aa) were used in the SOG/SOS fusion proteins: 5 aa (5′-GSSGG-3′); 73 aa (5′-GSGSAGGSAGGSAGGSAGGSAGGSAGGSADGSAGGSAGGSAGGSAGGSAGGSAGGSAGGSAGGSAGGSAGGSR-3′); and 133 aa (5′-GSGSAGGSAGGSAGGSAGGSAGGSAGGSAGGSAGGSAGGSAGGSAGGSAGGSAGGSAGGSAGGSAGGSAGGSAGGSAGGSAGGSAGGSAGGSAGGSAGGSAGGSAGGSAGGSAGGSAGGSAGGSAGGSAGGSR-3′). Constructs are listed in Supplementary Table 1 . Proteins were purified with the Ni-NTA purification system (Qiagen). Sample concentrations were quantified using the absorbance measurements of SOG and SOS and their extinction coefficients [12] , [13] . STET experiments were performed with fluorescence microscopy (see the Imaging section for details) or a 450±20-nm blue LED followed by fluorescence spectroscopy (see STET specificity section for details). Under the illumination conditions used, the photobleaching of SOS is negligible in the absence of SOG ( Fig. 4a ; Supplementary Fig. 9 ). STET specificity To demonstrate the specificity of IFP SOS and its cofactor BV, various ROS were added to 1 μM of SOS ( Fig. 2 ) or 50 μM of BV ( Fig. 3 ) in a reaction volume of 100 μl. Superoxide (O 2 · − ) was generated either with 1 mM of KO 2 or by reacting 1 m M of xanthine with 10 mU of xanthine oxidase. H 2 O 2 or sodium hypochlorite (NaClO) was added directly to the IFP or BV solution at a final concentration of 1 mM. To generate hydroxyl radical (·HO) via the Fenton reaction, 0.1 mM of Fe 2+ (from FeSO 4 ) was mixed with 1 mM of H 2 O 2 . To generate singlet oxygen ( 1 O 2 ) chemically, 1 mM of H 2 O 2 and 1mM of NaClO were mixed and added to the IFP or BV solution. To generate 1 O 2 photochemically, 10 μM of perinaphthenone was added to the IFP or BV solution. The reaction mixture was then illuminated with a 450±20-nm blue LED (Innovations in Optics, Woburn, MA) at an intensity of~\n50 mW cm −2 . The fluorescence emission (for SOS) and absorbance (for BV) spectra were measured at 25 °C at different time points. To further demonstrate specificity towards 1 O 2 , STET experiments using a mixture of 1 μM of SOG and 1 μM of SOS in a final volume of 100 μl were performed in the presence of various ROS quenchers ( Fig. 4 ). Three ROS quenchers were used: 1 U of SOD, 100 mU of catalase and 1 m M of GSH. The reaction mixture was illuminated with the 450±20-nm blue LED at ~\n50 mW cm −2 . Fluorescence emission spectra of SOS were obtained at different time points. All reactions and spectroscopic measurements were performed in phosphate-buffered saline buffer at pH 7.4. The absorbance and fluorescence emission spectra were obtained using the Tecan Infinite M1000 microplate reader. All chemicals were purchased from Sigma-Aldrich, except for xanthine (Calbiochem) and xanthine oxidase (Roche). Yeast strains and plasmids S. cerevisiae BY4741 ( Mat a his3 Δ 1 leu 2Δ 0 met15 Δ 0 ura3 Δ 0 ) was used as the parent strain. A haem oxygenase-1 ( HO1 ) human gene, flanked by the yeast TEF1 promoter and CYC1 terminator, was integrated into the his3 locus of BY4741 by homologous recombination to generate yTLT027. Heterologous expression of haem oxygenase-1 produces IFP’s cofactor, BV. All S. cerevisiae strains used in this study were derived from yTLT027. For expression of SOG and SOS fusion proteins, the high-copy episomal vectors p424TEF and p426TEF (from ATCC) were used. Both vectors carry the yeast TEF1 promoter and CYC1 terminator. DNA sequences encoding a miniSOG (miniSOG, 0.33 kb) and IFP1.4 (0.96 kb) were amplified from pcDNA3.1 vectors that carried the mammalian codon-optimized genes. The yeast genes MDM34 (1.4 kb), MMM1 (1.3 kb), MDM32 (1.9 kb), MGM101 (0.8 kb) and the pre-sequence of TOM70 (first 31 N-terminal residues) were individually PCR-amplified from the genomic DNA isolated from BY4741. An oligonucleotide-mediated recombination method was used to create fusion proteins of miniSOG or IFP1.4 (at the C terminus) with the above yeast genes directly in yeast cells to give Mmm1–SOG, Mdm34–SOS, Mgm101–SOS and Tom70–SOS. An additional fusion protein, SOS–Mdm34, was created by fusing IFP to the N terminus of Mdm34. All fusion proteins were flanked by Bam HI and Xho I restriction sites on the vectors. An eight-residue peptide spacer (GDGAGLIN) was inserted between the fusion partners. The nucleotide sequence of the peptide spacer contains a PacI restriction site (5′-ggtgacggtgctggtttaattaac-3′), allowing the swapping of fusion partners. The fusion proteins containing SOG were expressed with p426TEF, whereas those containing SOS were expressed with p424TEF. The constructs used in this study are listed in Supplementary Table 1 . Yeast growth Yeast YPD medium containing 1% Bacto-yeast extract, 2% Bacto-peptone and 2% dextrose was used to grow BY4741 and yTLT027. Synthetic dextrose medium containing 0.67% yeast nitrogen base, 2% dextrose and amino-acid dropout mix lacking tryptophan (for p424TEF selection) and uracil (for p426TEF selection) was used to select for transformants containing the fusion protein constructs. Yeast cultures were grown at 30 °C with constant shaking at 220 r.p.m. The yeast cells were harvested at the exponential growth phase (OD 0.5–1), fixed with 4% formaldehyde at room temperature for 45 min and washed twice. The cells were then concentrated by centrifugation and attached to the surface of an imaging cover glass coated with Concanavalin A. The edges of the cover glass were sealed with nail polish to prevent drying. Imaging Imaging of purified protein solutions and fixed yeast cells were performed with a Nikon Eclipse Ti inverted microscope with the Perfect Focus System. All instrument control and image acquisition were performed with home-written software in Python. Two diode lasers (488 nm at ~\n1 W cm −2 from Stradus, 488-50 and 642 nm at ~\n3 W cm −2 from Stradus 642-110; Vortran) were directly shuttered by the computer. A filter wheel was used to control the power of each laser. The two lasers were collimated into a telescopic optical path and focused to the back focal plane of the oil-immersion objective (Olympus × 100 UPlanSApo NA 1.4) on the microscope. A quad-band beam splitter zt405/488/561/640rpc (Chroma) and band-pass filters (ET525/50 for SOG, ET705/72 for SOS, Chroma) were used to separate the fluorescence signal. A two-colour split-view setup was used to simultaneously acquire SOG and SOS channels within a single- image frame. The emitted light was divided by a dichroic mirror (beam splitter 645 DCXR, Chroma), allowing the reflected light path to pass through the ET525/50 for SOG fluorescence and the transmitted light path to pass through the ET705/72 for SOS fluorescence. Both channels were projected on a single camera to produce a split image. The images were recorded with an electron multiplying CCD camera (Ixon DV897DCS-BV, Andor) at a frame rate of 1 Hz (1 s exposure time) for purified protein samples and 10 Hz (100 ms exposure time) for fixed yeast cells. Image analysis The images were analysed using ImageJ 1.42q (NIH http://rsbweb.nih.gov/ij/ ) and MATLAB (Mathworks). For each acquired image stack, the SOG and SOS channels were extracted from the split-view images and aligned using their corresponding bright-field images. After alignment, we identified candidate Mmm1 puncta from the SOG channel. For each punctum, we defined the corresponding overlapping SOS signal. For each pixel within the overlapping SOS signals, we analysed the loss in fluorescence over the experiment’s time course (typically 5 s). The pixel with the highest loss in SOS fluorescence was defined as the center. Drifting, and hence displacement of the center, was uncommon over the time course. As such, pixel-by-pixel alignment was usually not necessary. The signal loss of the immediate neighbour pixels was similar to that of the center ( Supplementary Fig. 10 ), rendering pixel-by-pixel calculation of STET signals unnecessary as well. Besides, pixel-by-pixel characterization of STET is subject to large fluctuations in fluorescence intensities. Hence, the signal loss of the center pixel and that of the surrounding 8 pixels (that is, a 3 × 3 region) were averaged for each Mmm1 punctum candidate. This average signal loss was used to determine the STET for the punctum. Only puncta with comparable area and SOG fluorescence intensity were analysed for their corresponding SOS intensity loss. At least five Mmm1 puncta were analysed per sample. Derivation of STET signal In our system, SOS is irreversibly bleached by singlet oxygen, that is, The mass action kinetics of the above reaction is described as: The mass balance of SOS is given by: Substitute (3) into (2): Here, [ 1 O 2 ] is the concentration of singlet oxygen at the site of SOS. In our STET results, the natural logarithm of normalized fluorescence intensity of SOS at different times can be well-fitted by a linear equation: y =− αt . The first-order kinetics in STET with respect to SOS implies constant singlet oxygen generation over the time course of experiments (that is, [ 1 O 2 ] is constant over time). Under such conditions, the solution of (4) is: where c= [ 1 O 2 ]. Taking the natural logarithm: The STET signal in this study is obtained from fitting the natural logarithm of normalized SOS fluorescence to a linear equation y =− αt . Comparing this to (6), α = kc , where c is governed by diffusion of 1 O 2 and is therefore dependent on the distance between SOG and SOS. The quantitative relationship between the STET signal and intermolecular distance should be the subject of future studies. How to cite this article : To, T.-L. et al . Singlet oxygen triplet energy transfer-based imaging technology for mapping protein–protein proximity in intact cells. Nat. Commun. 5:4072 doi: 10.1038/ncomms5072 (2014).